Growth and modelling of spherical crystalline morphologies of molecular materials Crystalline, yet smooth, sphere-like morphologies of small molecular compounds are desirable in a wide range of applications but are very challenging to obtain using common growth techniques, where either amorphous films or faceted crystallites are the norm. Here we show solvent-free, guard flow-assisted organic vapour jet printing of non-faceted, crystalline microspheroids of archetypal small molecular materials used in organic electronic applications. We demonstrate how process parameters control the size distribution of the spheroids and propose an analytical model and a phase diagram predicting the surface morphology evolution of different molecules based on processing conditions, coupled with the thermophysical and mechanical properties of the molecules. This experimental approach opens a path for exciting applications of small molecular organic compounds in optical coatings, textured surfaces with controlled wettability, pharmaceutical and food substance printing and others, where thick organic films and particles with high surface area are needed. Micro- and nanostructures based on small molecular materials have many promising applications: in optoelectronic devices with unique charge and light-transfer properties [1] , [2] , [3] , in sensors and in the pharmaceutical [4] and food industries. Spherical nanoparticles are useful building blocks in many fields, including photonics [5] , pharmaceuticals, surfaces with controlled wettability [6] , [7] and others. Challenges in scaling up and broadening their applications include the limited set of materials from which they have been made, and the ability to directly attach these particles to any desired surface. Achieving sphere-like morphologies using small molecular compounds is nearly impossible using common techniques, such as precipitation from solution [8] , aerosol-coating [9] or vacuum thermal evaporation (VTE). The traditional methods either yield smooth amorphous or faceted crystalline particles. Among vapour-based film growth techniques, VTE is one of the most widely implemented methods to fabricate small molecular organic thin films. In this method, the material is evaporated from a resistively heated boat under high vacuum (<10 −7 Torr) [10] . The evaporated molecules are ballistically transported to the substrate where they are adsorbed through van der Waals forces. In well-controlled conditions, quasi-epitaxial growth can persist for several monolayers, after which strain relaxation results in pronounced stacking defects [11] . Most of the organic thin film growths by VTE result in amorphous or nanocrystalline morphologies, while the substrate is usually heated in order to enhance crystallinity. Substrate templating involves using thin crystalline films of small molecular organic materials [12] , [13] or thin membranes of graphene [14] as seed layers. The degree of vapour saturation of organic material at the substrate is an important parameter that determines film morphology. Yao and colleagues [8] , for instance, have demonstrated the growth of single-crystal tris(8-hydroxyquinoline)aluminum (Alq 3 ) nanowires using adsorbent-assisted physical vapour deposition, where the degree of saturation of Alq 3 can be controlled via adsorbents in the vapour phase. Huang et al . [15] developed a method for the micropatterned growth of iron phthalocyanine (FePc) nanofibre arrays using VTE by controlling the surface energy and temperature of the substrate, where a grain-like (in-plane) morphology was obtained on Si surfaces (higher surface energy) and a fibre-like (out-of-plane) morphology was obtained on silver surfaces (lower surface energy) within a certain range of substrate temperatures. Chiu et al . [3] have used a vapour condensation method for the growth of Alq 3 nanowires. Organic vapour phase deposition is an alternative vapour growth technique, based on subliming small molecular organic materials into a stream of inert carrier gas under a low-vacuum environment [16] . In organic vapour phase deposition, the crystalline domain size is controlled by adjusting the substrate temperature, carrier gas flow rate and chamber pressure. Using this method, Yang et al . [1] showed controlled growth of ordered bulk heterojunction photovoltaic cells, where the electron donor layer of copper phthalocyanine exhibited a continuous wetting layer, with short needle-like crystals grown on top. Organic vapour jet printing (OVJP) [17] mixes organic vapour with an inert carrier gas, ejecting the mixture at high velocity (on the order of 100 m s −1 ) through a nozzle on a cold substrate, where the organic material selectively condenses. This approach enables direct, solvent-free, additive patterning of small molecular organic materials and is typically performed under a low vacuum of 0.1–10 Torr. In guard flow-enhanced organic vapour jet printing (GF-OVJP) [18] , [19] , [20] , the primary inner jet of organic vapour and carrier gas is hydrodynamically focused by an annular, coaxial jet of inert gas (guard flow). GF-OVJP enables printing at lower vacuum levels than OVJP and even under ambient conditions. 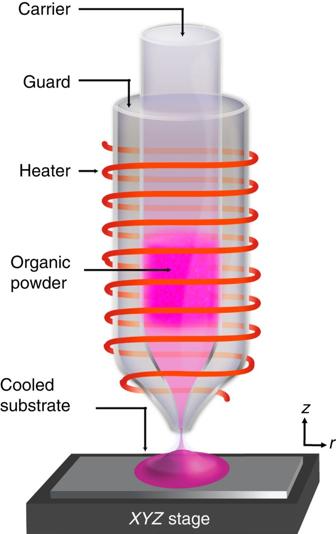Figure 1: Schematic of GF-OVJP system. Powdered organic material is loaded in the heated sublimation zone. The evaporated molecules are jetted on the cooled substrate using an inert carrier gas, surrounded with inert guard flow gas. Figure 1 demonstrates the GF-OVJP working principle. Process parameters include nozzle–substrate separation distance, evaporation (sublimation) zone temperature, substrate temperature, carrier gas flow rate and guard gas flow rate. Powdered organic material is loaded in the sublimation zone and heated, while carrier and guard gas rates are held constant. The hot evaporated material is jetted on the cooled substrate at flow velocities of ~200 m s −1 , enabling high local deposition rate of tens of nanometres per second. This approach is particularly interesting for a broad set of applications, not only because of the additional morphological control but also because of its ability to generate relatively thick (>500 nm) and large area deposits, while also enabling additive patterning with high material-utilization efficiency. Figure 1: Schematic of GF-OVJP system. Powdered organic material is loaded in the heated sublimation zone. The evaporated molecules are jetted on the cooled substrate using an inert carrier gas, surrounded with inert guard flow gas. Full size image Here we use GF-OVJP to generate the growth of variable aspect ratio microfeatures that are attached to the substrate and exhibit crystallinity without faceting. Below we describe some of the growth modes and propose a model that can quantitatively predict surface morphology in small molecular organic films. We demonstrate the growth of continuous, non-faceted, crystalline microspheroids of archetypal small molecular organic semiconductor compounds— boron subphthalocyanine chloride (SubPc) and Alq 3 . Using a surface evolution framework of small molecular organic film growth, we present an analytical model to describe the highly kinetic and thermal aspect of GF-OVJP deposition. The model incorporates the thermophysical, structural and mechanical properties of the materials and is validated by observed morphologies. It can be used to predict nanostructured morphologies in films of different materials with known thermophysical and mechanical properties. Morphology evolution SubPc is an archetypal small organic material, commonly used as an electron donor material in organic photovoltaic cells. This molecule has a conical shape with an orthorhombic crystal structure [21] in the bulk phase. 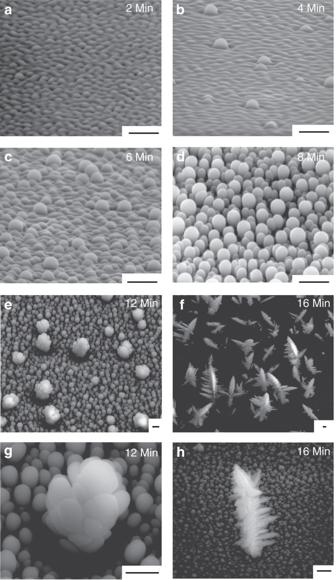Figure 2: Surface evolution of SubPc film. This film was continuously grown by GF-OVJP at evaporation temperature of 325 °C with dwell time durations of stationary nozzle above the substrate as indicated on the figures: (a) 2 min, (b) 4 min, (c) 6 min, (d) 8 min, (e) 12 min, (f) 16 min, (g) 12 min—enlarged, (h) 16 min—enlarged. Scale bar 1 μm. Alq3film growth resulted in similar surface evolution (Supplementary Fig. 5). Figure 2 shows the surface evolution of SubPc grown on (100) silicon using GF-OVJP at a source temperature of 325 °C. Smooth thin films are obtained up to a film thickness of ~200 nm, evolving into wavy, sinusoidal-like morphology upon further growth ( Fig. 2a ). Beyond a critical total thickness (~800 nm), the film evolves into a spheroidal, lobe-like morphology ( Fig. 2b–d ). From this point on, film thickness remains constant and only the lobes grow, eventually combining into fern-like microstructures ( Fig. 2e–h ). Figure 2: Surface evolution of SubPc film. This film was continuously grown by GF-OVJP at evaporation temperature of 325 °C with dwell time durations of stationary nozzle above the substrate as indicated on the figures: ( a ) 2 min, ( b ) 4 min, ( c ) 6 min, ( d ) 8 min, ( e ) 12 min, ( f ) 16 min, ( g ) 12 min—enlarged, ( h ) 16 min—enlarged. Scale bar 1 μm. Alq 3 film growth resulted in similar surface evolution ( Supplementary Fig. 5 ). Full size image Effect of process conditions To understand the role of vapour saturation on growth kinetics and morphology, the source temperature was varied, while keeping all the other process parameters constant. The resulting mean lobe diameter and diameter distribution width ( Fig. 3 ) decrease with an increase in source temperature. As evaporation source temperature increases, the partial pressure and concentration of organic material in the carrier gas jet increases; nucleation density (or number of nuclei per unit area) increases, in turn, with the concentration of organic admolecules. These denser nucleation sites act as surface perturbations, thus promoting smaller and more uniform lobe formation with higher source temperature. These trends are shown clearly in Fig. 3c . Further growth results in coarsening of the lobes, as shown in Fig. 3b . In this case, the experiment was performed at a constant source temperature of 310 °C, while the nozzle dwell time was varied. The coarsening can be explained by an Ostwald ripening mechanism ( Fig. 3d ), where large particles grow at the expense of smaller particles. In this case, there is a linear relation between the average particle diameter cubed and time, as expected by Ostwald theory [22] . Additional aspects of this phenomenon are discussed in Supplementary Note 1 . 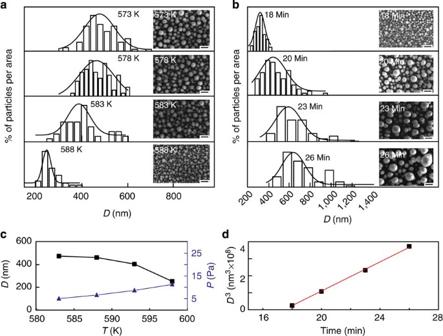Figure 3: Morphology control in GF-OVJP. (a) Distribution of lobe diameters for different source temperatures. Scale bar 1 μm. (b) Distribution of lobe diameters with time. Scale bar 1 μm. (c) Effect of temperature on average lobe diameters and partial pressure of the evaporating moleculesP(Pa) near the material source. (d) Lobe coarsening process plotted as cube of average lobe diameter versus time (black data points) with linear fit (red line). Figure 3: Morphology control in GF-OVJP. ( a ) Distribution of lobe diameters for different source temperatures. Scale bar 1 μm. ( b ) Distribution of lobe diameters with time. Scale bar 1 μm. ( c ) Effect of temperature on average lobe diameters and partial pressure of the evaporating molecules P (Pa) near the material source. ( d ) Lobe coarsening process plotted as cube of average lobe diameter versus time (black data points) with linear fit (red line). Full size image X-ray diffraction In situ X-ray diffraction (XRD) reveals that the films are polycrystalline throughout the growth ( Fig. 4a ). The linear dependence of peak height on growth time ( Supplementary Fig. 1 ) indicates that the lobes, as well as the wetting layer, are polycrystalline, and the degree of crystallinity does not change. Ex situ XRD was performed with the X-ray incidence angle below the critical angle (~0.1°) of the film containing the lobe structures ( Fig. 4b ), such that the diffraction beam probes only the top 10 nm of the deposit. Powder rings with uniformly distributed intensity were observed, suggesting that the lobes are highly polycrystalline throughout, without any preferred orientation. The average size of the crystallites is calculated to be ~50 nm using Scherrer’s equation [23] , while the lobes are ~500 nm in diameter, indicating that each lobe comprises number of crystallites. Measured peak positions are in very good agreement with those from reported bulk crystal structure of SubPc [21] , indicating that the crystal structure of the film as well as that of the lobes is similar to that of bulk SubPc, which was used as the evaporation source material. However, the lobes are non-faceted. This unusual growth modality can be understood in part by considering the balance of driving forces in the thin film growth. 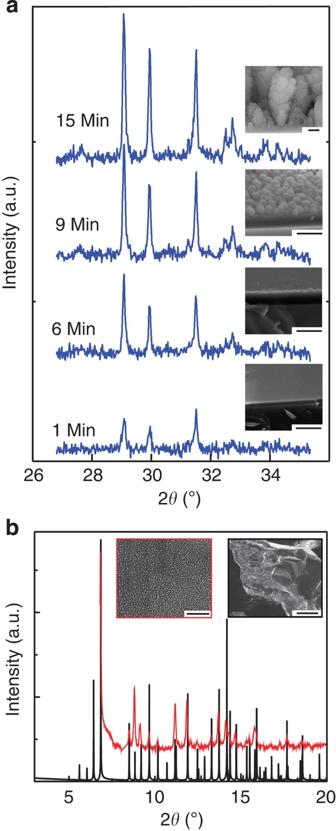Figure 4: XRD results. (a)In situXRD measurement during the film growth showed that the diffraction peak intensities continuously increase as a function of film thickness, regardless of the morphology of the film surface (smooth, wavy, lobes and ferns). Diffraction intensity data at four different film thicknesses (nozzle dwell time: 1, 6, 9 and 15 min) are shown, and the scanning elecrtron microscopy image insets describe the morphology of the film surface at each growth stage. Scale bar 1 μm. (b) Full 2θscan of deposit with lobe microstructure (red curve) and simulated powder diffraction pattern from its bulk structure21(black curve) showing good agreement between their peak positions. Inset depicts the micrographs of SubPc bulk powder and deposit. Scale bar 10 μm. Figure 4: XRD results. ( a ) In situ XRD measurement during the film growth showed that the diffraction peak intensities continuously increase as a function of film thickness, regardless of the morphology of the film surface (smooth, wavy, lobes and ferns). Diffraction intensity data at four different film thicknesses (nozzle dwell time: 1, 6, 9 and 15 min) are shown, and the scanning elecrtron microscopy image insets describe the morphology of the film surface at each growth stage. Scale bar 1 μm. ( b ) Full 2 θ scan of deposit with lobe microstructure (red curve) and simulated powder diffraction pattern from its bulk structure [21] (black curve) showing good agreement between their peak positions. Inset depicts the micrographs of SubPc bulk powder and deposit. Scale bar 10 μm. Full size image Significant surface perturbations in the film arise beyond a thickness of 200 nm. Unlike other vapour-based deposition methods, where the source of organic material is far from the substrate (usually 50 cm and more), in GF-OVJP, the jet temperature within 10 μm of the substrate reaches 200 °C. Consequently, the in-plane and out-of-plane thermal gradients in the film increase with film thickness because of the low thermal conductivity of organic materials (~0.1 W m −1 K −1 ) [24] , causing elastic strains in and out of the substrate plane. 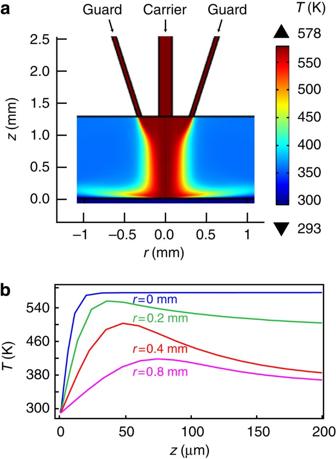Figure 5: Temperature distribution in the GF-OVJP system. (a) Temperature of jet exiting the nozzle and impinging on the substrate. (b) Temperature distribution across substrate–nozzle region at different radial positions. Figure 5a,b shows the thermal gradients occurring within a film grown by GF-OVJP. The wave-like surface perturbations obtained here are reminiscent of Stransky–Krastanov growth, usually occurring in inorganic materials because of substrate-film crystal mismatch, which leads to the formation of quantum dots and nanorods [25] . In the present case, the stresses originate from the thermal gradients within the film; therefore, significantly larger critical thicknesses are required to obtain the thermal stress needed to cause a three-dimensional (3D) surface formation. The evolution of a wavy surface instability into the observed spheroidal shapes depends on the balance between the energy relaxation of the thermally driven elastic strain in the film, and the energy cost of increasing the surface area, embodied by ref. 26 : Figure 5: Temperature distribution in the GF-OVJP system. ( a ) Temperature of jet exiting the nozzle and impinging on the substrate. ( b ) Temperature distribution across substrate–nozzle region at different radial positions. Full size image where G is the body free energy of the system per wavelength (J m −1 ); γ is the surface energy (J m −2 ); λ is the surface waviness wavelength (m); Y is material’s Young’s modulus (Pa); σ is the stress acting on the surface (Pa) and q is the amplitude of the perturbation (m). The perturbation is amplified when the wavelength λ exceeds a critical value, given by: where λ c is the critical wavelength beyond which the surface is no longer stable and 3D growth occurs. For the SubPc system, the measured surface energy is 44.7 mJ m −2 ; the estimated Young’s modulus (from other phthalocyanine materials) [27] is ~5 GPa. The thermal expansion coefficient of SubPc is 1.4 × 10 −4 K −1 in the amorphous phase and 6.5 × 10 −4 K −1 in the crystalline phase (see Methods section on thermal expansion coefficient measurement and Supplementary Fig. 2 ). For 800 nm film thickness, temperature differences both in-plane and out-of-plane of the film can reach tens of degrees ( Fig. 1b ), resulting in thermal stresses acting on the surface being on the order of tens to hundreds MPa (depending on deposition conditions). For these values, the critical wavelength is on the order of 100 nm, in good agreement with experimentally observed critical wavelength for SubPc ( Fig. 6a ). As deposition continues, film thickness increases, and so does the amplitude of the waviness. When lobes start to form, the film thickness does not increase anymore and only spheres are growing. 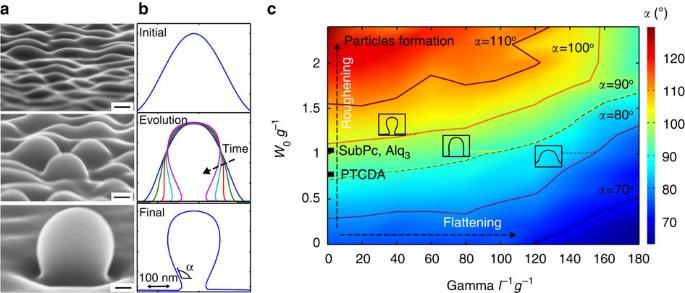Figure 6: Surface evolution simulation. (a) Evolution of surface from wave to lobe shape. Scale bar 1 μm. (b) Simulated evolution from wave into lobe shape modelled using finite element difference approach. (c) Contour plot of possible final geometries with respect to deviation from surface, as a function of dimensionless ratio of material surface energy gamma and initial maximal elastic energyW0to material bulk energyg(gas–solid phase transition enthalpy in this case).l, characteristic length-scale of interest, taken here as 1 nm. Figure 6: Surface evolution simulation. ( a ) Evolution of surface from wave to lobe shape. Scale bar 1 μm. ( b ) Simulated evolution from wave into lobe shape modelled using finite element difference approach. ( c ) Contour plot of possible final geometries with respect to deviation from surface, as a function of dimensionless ratio of material surface energy gamma and initial maximal elastic energy W 0 to material bulk energy g (gas–solid phase transition enthalpy in this case). l , characteristic length-scale of interest, taken here as 1 nm. Full size image To model the surface evolution, we start with an equation describing the driving force acting on a given surface element during growth and under mechanical stress [26] : where: P f —driving force (N m −2 ); γ —surface energy (J m −2 ), K —surface curvature (m −1 ); g —phase transition enthalpy (J m −3 ); and W —elastic strain energy (J m −3 ). The relation between the driving force and velocity normal to the surface of a surface element is where v n is the surface element velocity (m s −1 ) and L is surface element mobility (m 2 s kg −1 ). Then, the velocity of each surface point during the evolution can be recalculated with each time step according to the new surface geometry and the resulting driving force (see Supplementary Figs 3 and 4 and Supplementary Note 2 for details of the model). The surface strain energy at a nodal point i, W i is approximated via Equation (5), where the maximum strain energy is at the surface valleys: where r is a dimensionless constant matched to surface waviness and is the elemental deviation from the average surface height . Figure 6b shows the predicted morphological evolution at different time steps. The mechanism for spheroidal morphology formation obtained using this analytical model is in good agreement with the experiments. The process of surface evolution happens simultaneously with growth and film-annealing, which is the main reason for the observed phenomenon of obtaining crystalline, yet smooth and spherical microstructures. Figure 6c is a contour plot of the resulting morphologies where the figure of merit is a deviation angle α from the surface. Different morphologies and their associated α values are obtained by varying the dimensionless numbers W 0 g −1 and γ l −1 g −1 ), relating the surface energy γ ( gamma in the Fig. 6c ) and initial maximum elastic energy W 0 to phase transition enthalpy g , respectively. Here l (m) is a characteristic scale of interest. A deviation angle greater than 90 degrees will lead to spheroidal morphologies, while deviation angles close to 90 degrees will result in platelet-like morphology. Deviations less than 90 degrees will result in a less wavy morphology with a tendency towards surface flattening. Surface energy and phase transition enthalpy are intrinsic material properties, while elastic strain energy is calculated from both intrinsic mechanical properties and deposition parameters (for example, inasmuch as they determine the degree of thermal expansion and strain). There is thus a trade-off between surface and elastic energies; while high surface energy will flatten the films, low surface energy will result in lobe formation. The model, therefore, can be used to describe morphologies of other organic materials under different processing conditions and provide a foundation for understanding microstructure formation and evolution. As an example, while Alq 3 films deposited by GF-OVJP show identical spherical morphologies ( Supplementary Fig. 5 ) because of similar intrinsic properties and process conditions, organic molecules with high anisotropy in molecular shape and mechanical properties, such as Perylene-3,4,9,10-tetracarboxylic dianhydride (PTCDA) evolve a platelet-like morphology ( Supplementary Fig. 5 ). All samples in the current study were deposited on (100) silicon. Similar microstructures were obtained on different orientations of silicon: (110) and (111), as well as on Si (100) substrate coated with 100-nm Al, indicating that the obtained microstructures are a result of temperature profiles in the substrates and the film coatings, rather than related to the crystal structure of the substrate. We observed new spheroidal crystalline (‘lobe’-like) microstructures comprising small organic molecules, with controllable and scalable sizes (100 nm to 1 μm), when grown by organic vapour jet printing. Initially, the film surface forms wave-like features with a characteristic wavelength, which evolve into lobes. XRD indicated these lobes to be crystalline, despite their non-faceted shape. A model was developed for surface evolution that can be applied for the prediction and quantitative understanding of small molecular-based film morphologies obtained via different growth techniques and conditions. For example, we showed that some organic materials will not exhibit lobe growth but instead will show platelet-like features, confirmed by the experiment. The deposition approach discussed here opens a new path for applications of small organic molecular materials where microstructural features of interest are on the order of hundreds of nanometres. These include optoelectronic device applications with high charge carrier mobility and exciton diffusion length [28] , antireflection coatings [29] , hydrophobic/oleophobic/omniphobic textured surfaces ( Supplementary Fig. 6 ), as well as the printing of pharmaceutical and food substances [30] , where thick organic films with high surface area are needed. Film fabrication All organic materials were purchased at sublimed grade purity from Luminescence Technology Corp. and deposited with no further purification. SubPc, Alq 3 and PTCDA were sublimed grade. All samples were deposited on Si (100) wafers. These were cleaned using ultrasonication in detergent solution and deionized water followed by heated acetone, trichloroethylene and isopropanol for 10 min each. Substrates were then placed in boiling isopropanol for 5 min and dried in pure nitrogen gas before film deposition. In order to check the effect of Si substrate orientation and remove native silicon oxide, the substrates were etched in hydrofluoric acid for 2 min before deposition. GF-OVJP process parameters The GF-OVJP nozzles used in this study were constructed from two coaxial glass tubes of 0.5′′ and 0.75′′ outer diameters, fused at one end and pulled at the other to form concentric nozzle tips of 200 and 700 μm internal diameters. The inert carrier gas and evaporated organic were transported through the inner tube. The inner gas used was 99.99% pure nitrogen. The annular channel for the guard jet was found to be 100 μm wide and was angled at ~15° from the nozzle axis. The nozzle was cleaned with solvents, dried and wrapped with 36‐gauge heavy insulated tape heater (Omega Engineering, Inc.) with a power density of 8.6 W in −2 . The heating tape leads were connected to a temperature controller (Digi‐Sense Benchtop temperature controller, Cole‐Palmer Instruments Co.) and a 1/16′′-K‐type thermocouple was used to maintain the temperature of the source. The source consisted of 0.15 g of powder embedded in a quartz wool and placed in the heated source section of the inner tube. The carrier gas and guard jet flow rates were maintained using mass flow controllers (C100 MFC, Sierra Instruments). The process parameters that were kept constant are as follows: nozzle–substrate separation distance, 1 mm; substrate temperature, 20 °C; carrier gas flow rate, 100 sccm; and guard gas flow rate, 200 sccm. The process was performed in glove box purged with 99.99% pure N 2 . X-ray measurements For all X-ray measurements, standard timescans ( in situ ) or 2 θ scans ( ex situ ) were taken in the vertical scattering plane with a PILATUS 100-K pixel detector. In situ XRD experiments were conducted at the beamline X21 (wiggler source) of the National Synchrotron Light Source (NSLS) at Brookhaven National Laboratory with 10-keV X-ray energy. The detector was placed at a fixed 2 θ position, and the detector images were taken every second during the film growth. The detector covers about 7° of 2 θ angular range with 0.02° resolution. The ex situ measurements were carried out at Sector 13-BM-C (15 keV, bending magnet source) and Sector 33-ID-D (15 keV, undulator source) of the advanced photon source (APS) at the Argonne National Laboratory. X-ray reflectivity data were first measured with a typical θ –2 θ scan to determine the critical angle for total external reflection, and full 2 θ scans were performed twice for each sample, with the X-ray incidence angle above and below the critical angle. Microscopy An FEI Nova 200 Nanolab scanning electron microscope with accelerating voltage of 5–10 kV and current 0.1–0.5 nA was used to obtain the surface morphology images. Thermal expansion coefficient measurement Spectroscopic ellipsometry was used to measure the time-dependent thickness changes exhibited by the samples when heating from room temperature to temperature, T , of 250 °C, at 1 °C min −1 , using a variable angle spectrometric ellipsometer (M-2000, J.A. Woollam Co.) equipped with an Instec heating stage. The measurements were performed at a fixed angle of 70°. More details are given in Supplementary Fig. 2 . Surface energy measurements of SubPc films For surface energy measurements, a GF-OVJP-deposited 100-μm film of SubPc was used. All contact angles were measured by advancing angle with ~2 μl of liquid on the surface (Ramé-Hart 200-F1 goniometer). Water was used as a polar liquid for polar surface energy measurement and methyl iodide (CH 2 I 2 ) was used as a nonpolar liquid for dispersive surface energy measurement. Modelling The COMSOL Multiphysics 4.3a software with a fluid dynamics module was used for temperature and flow profiles, and a mechanical module for stress calculations. For surface evolution modelling, Matlab_R2012b was used. A Finite element approach was used, as described in Supplementary Fig. 3 and Supplementary Note 2 . How to cite this article: Shalev, O. et al . Growth and modelling of spherical crystalline morphologies of molecular materials. Nat. Commun. 5:5204 doi: 10.1038/ncomms6204 (2014).